ERK7 regulates ciliogenesis by phosphorylating the actin regulator CapZIP in cooperation with Dishevelled Cilia are essential for embryogenesis and maintenance of homeostasis, but little is known about the signalling pathways that regulate ciliogenesis. Here, we identify ERK7, an atypical mitogen-activated protein kinase, as a key regulator of ciliogenesis. ERK7 is strongly expressed in ciliated tissues of Xenopus embryos. ERK7 knockdown markedly diminishes both the number and the length of cilia in multiciliated cells, and it inhibits the apical migration of basal bodies. Moreover, ERK7 knockdown results in a loss of the apical actin meshwork, which is required for the proper migration of basal bodies. We find that the actin regulator CapZIP, which has been shown to regulate ciliogenesis in a phosphorylation-dependent manner, is an ERK7 substrate, and that Dishevelled, which has also been shown to regulate ciliogenesis, facilitates ERK7 phosphorylation of CapZIP through binding to both ERK7 and CapZIP. Collectively, these results identify an ERK7/Dishevelled/CapZIP axis that regulates ciliogenesis. The mitogen-activated protein (MAP) kinase family plays an essential role in various processes such as cell proliferation, responses to stress and differentiation [1] . In vertebrates, there are 14 members of the MAP kinase family [2] . Among these, ERK7 (also known as ERK8 or MAPK15) is the most recently identified member, and is evolutionarily conserved throughout the animal kingdom. ERK7 undergoes autophosphorylation and is constitutively active [3] . Previous studies in cultured cells have shown that ERK7 is involved in the protection of genomic integrity, response to amino-acid starvation and autophagy [4] , [5] , [6] . However, its function in vivo remains largely unknown. Cilia, which are microtubule-based organelles, exert various important functions, such as the generation of fluid flow, sensing of extracellular stimuli and Hedgehog signal transduction, and they are essential for embryogenesis and the maintenance of homeostasis [7] , [8] . Defects in cilia cause a wide range of disorders, known as ciliopathy [9] . Ciliogenesis is a multistep process that includes basal body migration [7] . Although structural components of cilia and transcription factors that are essential for ciliogenesis have been extensively investigated, little is known about signalling pathways that regulate ciliogenesis. In this study, we aimed to identify the physiological function of ERK7 during embryogenesis using Xenopus embryos. Our results show that ERK7 is required for ciliogenesis. They further demonstrate that ERK7 is required for basal body migration and apical actin organization in multiciliated cells (MCCs). Mechanistically, ERK7 phosphorylates the actin regulator CapZIP that regulates ciliogenesis in a phosphorylation-dependent manner [10] . Moreover, Dishevelled (Dvl), which also regulates ciliogenesis [11] , facilitates ERK7 phosphorylation of CapZIP by binding to both ERK7 and CapZIP. These results identify an ERK7/Dvl/CapZIP axis that regulates ciliogenesis. Expression patterns of ERK7 during Xenopus development Whole-mount in situ hybridization showed maternal expression of ERK7 in the animal hemisphere ( Supplementary Fig. 1a ). Interestingly, zygotic ERK7 messenger RNA (mRNA) was highly expressed in ciliated tissues. At stage 12 (late gastrula), ERK7 expression was detected in the dorsal involuting marginal zone (DIMZ; Fig. 1a ). Costaining of ERK7 with FoxJ1 , which is expressed in the DIMZ [12] , showed that the region expressing ERK7 overlapped with the region expressing FoxJ1 ( Supplementary Fig. 1b ), confirming that ERK7 is expressed in the DIMZ. After involution through the blastopore, DIMZ forms the gastrocoel roof plate (GRP), on which motile monociliated cells are located [13] . ERK7 was expressed in the GRP at stage 16 (neurula stage; Fig. 1b ). At stage 25 (early tailbud stage) and stage 33/34 (late tailbud stage), ERK7 was expressed in the floor plate, cloaca and ear vesicle ( Fig. 1a and Supplementary Fig. 1c ), all of which are ciliated tissues. At stage 33/34 (late tailbud stage), ERK7 expression was also detected in nephrostomes, which are ciliated funnels. In addition, a salt-and-pepper expression pattern of ERK7 was observed in the epidermis ( Fig. 1a ). This expression pattern was observed at stage 13 and thereafter ( Fig. 1c ). In the Xenopus epidermis, four types of cells, alpha-ionocytes, beta-ionocytes, small secretory cells and MCCs, are distributed in a salt-and-pepper pattern [14] , [15] , [16] , [17] , [18] , [19] . MCCs bear many cilia on their surface, and therefore, they can be detected by immunostaining with an antibody against acetylated α-tubulin (a marker of cilia). To determine whether ERK7 is expressed in MCCs on the epidermis, we combined ERK7 in situ hybridization with acetylated α-tubulin immunostaining. The in situ staining of ERK7 on the epidermis completely coincided with acetylated α-tubulin immunostaining ( Fig. 1d ), indicating that ERK7 is specifically expressed in MCCs on the epidermis. No detectable signal was observed with the sense probe ( Supplementary Fig. 1d ). These results indicate that ERK7 is specifically expressed in ciliated tissues during Xenopus development. 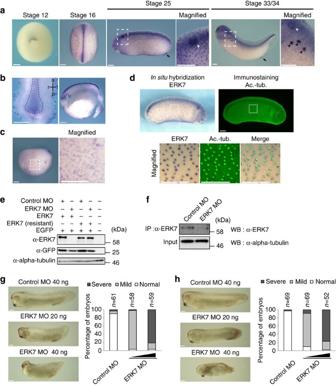Figure 1: Expression patterns ofERK7and knockdown phenotypes. (a–d) Whole-mountin situhybridization analysis ofERK7expression. Magnified images show regions outlined with white dashed lines. (a) The embryos at stage 12 (vegetal view), stage 16 (dorsal view), stage 25 and stage 33/34. Black arrows, cloaca; white arrowheads, ear vesicle; black arrowheads, nephrostomes. (b) The dorsal explant (left panel) and sagittal section (right panel) of the stage 16 embryo. The GRP is outlined by the black dotted line or indicated by the open arrowhead. a, anterior; l, left; p, posterior; r, right. (c) An embryo at stage 13 (lateral view). (d) Whole-mountin situhybridization ofERK7followed by immunostaining with anti-acetylated α-tubulin (Ac.-tub., green). (e,f) The efficiency of ERK7 MO. (e) The indicated sets of MO (10 ng per cell) and mRNA (500 pg per cell) were injected into the two blastomeres at the two-cell stage, and the embryos were harvested at stage 10.5. EGFP mRNA (100 pg per cell) was used as an injection control. (f) Each MO (10 ng per cell) was injected into the animal region of four blastomeres at the four-cell stage. Injected embryos were harvested at stage 33/34. Endogenous ERK7 protein was concentrated by immunoprecipitation from embryo lysates. (g,h) Knockdown experiments of ERK7. Control MO (20 ng per cell) or ERK7 MO (10 or 20 ng per cell) was injected into the dorsal (g) or ventral (h) marginal region of two blastomeres at the four-cell stage. The injected embryos were fixed and observed at stage 33/34. The phenotypes were classified into three groups (severe, mild or normal) according to the extent of the defects in head morphology (g) or body length (h). Scale bars, 300 μm. Figure 1: Expression patterns of ERK7 and knockdown phenotypes. ( a – d ) Whole-mount in situ hybridization analysis of ERK7 expression. Magnified images show regions outlined with white dashed lines. ( a ) The embryos at stage 12 (vegetal view), stage 16 (dorsal view), stage 25 and stage 33/34. Black arrows, cloaca; white arrowheads, ear vesicle; black arrowheads, nephrostomes. ( b ) The dorsal explant (left panel) and sagittal section (right panel) of the stage 16 embryo. The GRP is outlined by the black dotted line or indicated by the open arrowhead. a, anterior; l, left; p, posterior; r, right. ( c ) An embryo at stage 13 (lateral view). ( d ) Whole-mount in situ hybridization of ERK7 followed by immunostaining with anti-acetylated α-tubulin (Ac.-tub., green). ( e , f ) The efficiency of ERK7 MO. ( e ) The indicated sets of MO (10 ng per cell) and mRNA (500 pg per cell) were injected into the two blastomeres at the two-cell stage, and the embryos were harvested at stage 10.5. EGFP mRNA (100 pg per cell) was used as an injection control. ( f ) Each MO (10 ng per cell) was injected into the animal region of four blastomeres at the four-cell stage. Injected embryos were harvested at stage 33/34. Endogenous ERK7 protein was concentrated by immunoprecipitation from embryo lysates. ( g , h ) Knockdown experiments of ERK7. Control MO (20 ng per cell) or ERK7 MO (10 or 20 ng per cell) was injected into the dorsal ( g ) or ventral ( h ) marginal region of two blastomeres at the four-cell stage. The injected embryos were fixed and observed at stage 33/34. The phenotypes were classified into three groups (severe, mild or normal) according to the extent of the defects in head morphology ( g ) or body length ( h ). Scale bars, 300 μm. Full size image ERK7 is required for ciliogenesis To examine ERK7 function, we performed knockdown experiments using an antisense morpholino oligonucleotide (MO), which was designed to block the translation of ERK7. We also generated an antibody against Xenopus ERK7. Immunoblotting analysis showed that ERK7 MO inhibited the translation of exogenous ERK7 ( Fig. 1e ), and significantly reduced endogenous ERK7 protein levels ( Fig. 1f ). Embryos that had been dorsally injected with ERK7 MO displayed reduced head structures, close-set eyes and dorsal curvature ( Fig. 1g ). On the other hand, embryos that had been ventrally injected with ERK7 MO displayed loss of fin ( Fig. 1h ). A higher dose of ERK7 MO resulted in the inhibition of antero-posterior axis elongation and breakdown of the epidermis, which resulted in exposure of the inner tissues to the outer environment ( Fig. 1h ). In fact, the higher dose of ERK7 MO caused a loss of epidermal cells such as small secretory cells ( Supplementary Fig. 2 ). ERK7 knockdown with a second non-overlapping ERK7 MO caused defects similar to those caused by the first MO in both dorsal and ventral injections ( Supplementary Fig. 3a,b ). We noticed that ERK7 knockdown in the epidermis abrogated the hovering movement of embryos, which is driven by MCC-generated fluid flow ( Supplementary Movies 1 and 2 ). To directly monitor the fluid flow, we added fluorescent beads to the culture media and monitored the bead movement. While beads moved fast in a cranio–caudal direction in control embryos as previously reported [20] , beads hardly moved in ERK7 morphants ( Fig. 2a,b and Supplementary Movies 3 and 4 ). These results indicate that ERK7 knockdown results in the loss of MCC-generated fluid flow. 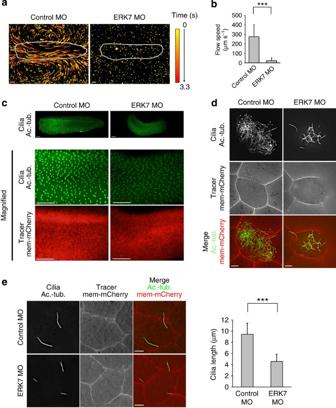Figure 2: ERK7 is required for ciliogenesis. (a) The trajectories of fluorescent beads are shown in a colour gradient (see colour bar). Each MO (10 ng per cell) was injected into the animal region of four blastomeres at the four-cell stage. White lines indicate an outline of the embryo. SeeSupplementary Movies 3 and 4. Scale bars, 300 μm. (b) The flow velocity of the beads was measured using ImageJ. Error bars represent the s.d. of 90 beads from nine embryo movies for each condition. ***P<0.001 by thet-test. (c–e) Immunostaining with anti-acetylated-α-tubulin (Ac.-tub) to visualize cilia (green). As a tracer, membrane-targeted (mem)-mCherry (red) was used. (c,d) Each MO (10 ng per cell) was injected into the animal region of four blastomeres at the four-cell stage. The injected embryos were fixed at stage 35/36. (c) Whole embryos. Scale bars, 300 μm. (d) Multicilia on MCCs. Scale bars, 5 μm. (e) Cilia on the GRP. Each MO (15 ng/cell) was injected into the dorsal marginal region of two blastomeres at the four-cell stage. The right graph shows the average length of cilia on the GRP (control MO,n=62 from five dorsal explants; ERK7 MO,n=97 from five dorsal explants). Error bars represent the s.d. Scale bars, 5 μm. ***P<0.001 by thet-test. Figure 2: ERK7 is required for ciliogenesis. ( a ) The trajectories of fluorescent beads are shown in a colour gradient (see colour bar). Each MO (10 ng per cell) was injected into the animal region of four blastomeres at the four-cell stage. White lines indicate an outline of the embryo. See Supplementary Movies 3 and 4 . Scale bars, 300 μm. ( b ) The flow velocity of the beads was measured using ImageJ. Error bars represent the s.d. of 90 beads from nine embryo movies for each condition. *** P <0.001 by the t -test. ( c – e ) Immunostaining with anti-acetylated-α-tubulin (Ac.-tub) to visualize cilia (green). As a tracer, membrane-targeted (mem)-mCherry (red) was used. ( c , d ) Each MO (10 ng per cell) was injected into the animal region of four blastomeres at the four-cell stage. The injected embryos were fixed at stage 35/36. ( c ) Whole embryos. Scale bars, 300 μm. ( d ) Multicilia on MCCs. Scale bars, 5 μm. ( e ) Cilia on the GRP. Each MO (15 ng/cell) was injected into the dorsal marginal region of two blastomeres at the four-cell stage. The right graph shows the average length of cilia on the GRP (control MO, n =62 from five dorsal explants; ERK7 MO, n =97 from five dorsal explants). Error bars represent the s.d. Scale bars, 5 μm. *** P <0.001 by the t -test. Full size image Next, we performed immunostaining using an acetylated α-tubulin antibody to visualize the cilia. Although the staining intensity of each spot on the epidermis was drastically reduced in ERK7 morphants, the number of spots was comparable to that in control embryos ( Fig. 2c ). As each spot represents MCC, this result indicates that ERK7 knockdown does not affect the number of MCCs. Higher magnification images revealed that both the number of cilia and the length of the formed cilia were strikingly diminished in ERK7 morphants ( Fig. 2d ). Moreover, ciliary beating was lost in ERK7 morphants ( Supplementary Movies 5 and 6 ). Injection of the second non-overlapping ERK7 MO resulted in the same defects in ciliogenesis ( Supplementary Fig. 3c ). In addition, the defect in cilia formation in ERK7 morphants was significantly rescued by the injection of MO-resistant ERK7 mRNA ( Supplementary Fig. 4 ). These results indicate that ERK7 is required for the process of ciliogenesis but not for the specification of ciliated cells. We next examined whether ERK7 is required for ciliogenesis in the GRP. Motile monocilia are known to be located on the GRP [13] , which is the functional equivalent of the node in the mouse and Kupffer’s vesicle in zebrafish [21] , [22] , [23] . The GRP cilia were shorter in ERK7 morphants than in control embryos ( Fig. 2e and Supplementary Fig. 5a ), indicating that ERK7 regulates ciliogenesis in many ciliated tissues. The GRP cilia are known to be posteriorly polarized [13] . We then analysed the polarization of the GRP cilia. ERK7 knockdown disturbed the polarization of the GRP cilia ( Supplementary Fig. 5b–d ), indicating that ERK7 is important for the polarization of GRP cilia. The GRP cilia are important for left-right axis specification [13] . Thus, we analysed the expression of Pitx2c, which is asymmetrically expressed in the left lateral plate mesoderm [24] . ERK7 knockdown resulted in a loss of asymmetric Pitx2c expression in the left lateral plate mesoderm ( Supplementary Fig. 6 ), indicating that ERK7 is important for left-right axis specification. ERK7 expression is under the control of FoxJ1 The above results indicate that ERK7 is required for ciliogenesis and is specifically expressed in ciliated tissues. Thus, we examined the regulation of ERK7 expression. FoxJ1 , one of the forkhead family genes, is a master regulator of the motile ciliogenic programme [12] , [25] , and its spatial expression pattern [12] , [26] is very similar to that of ERK7 . In addition, we noticed that in the deposited microarray data [12] , ERK7 was among the genes that were upregulated by the injection of FoxJ1 under the condition of ectopic expression of a Notch intracellular domain (NICD), which caused a loss of MCCs in the skin [14] . Thus, we examined whether ERK7 expression is regulated by FoxJ1 . We injected FoxJ1 mRNA into four-cell-stage embryos and harvested the embryos at stage 13 to evaluate ERK7 expression. Quantitative reverse transcription (RT)–PCR analysis showed that overexpression of FoxJ1 strongly induced ERK7 expression ( Fig. 3a ). Next, we examined the effect of NICD on ERK7 expression. Animal caps were prepared at stage 10 and then harvested at the equivalent of stage 19–20 to analyse ERK7 expression. The analysis showed that overexpression of NICD, which acts upstream of FoxJ1 and suppresses FoxJ1 expression [27] , [28] , decreased ERK7 expression ( Fig. 3b ). In agreement with the deposited microarray data [12] , the overexpression of FoxJ1 increased ERK7 expression even in the presence of NICD ( Fig. 3b ). Furthermore, we examined the effect of FoxJ1 knockdown on ERK7 expression. FoxJ1 MO resulted in a drastic decrease in ERK7 expression levels ( Fig. 3c ). These results indicate that ERK7 expression is under the control of FoxJ1 , the master regulator of ciliogenesis. Next, we examined whether FoxJ1 expression is affected by ERK7 . The result showed that neither overexpression of ERK7 nor ERK7 MO affected the expression level of FoxJ1 ( Supplementary Fig. 7a,b ). Thus, the FoxJ1 expression level is not affected by ERK7 . 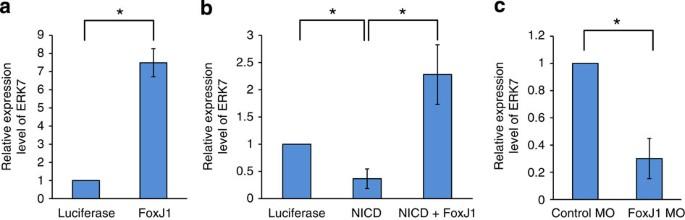Figure 3:ERK7expression is under the control of FoxJ1. (a–c) Quantitative RT–PCR analysis ofERK7expression levels. The average of three independent experiments is presented. The expression levels ofERK7were normalized to those ofODC. (a) Each mRNA (500 pg per cell) was injected into the animal region of four blastomeres at the four-cell stage. Injected embryos were harvested at stage 13 and assayed for ERK7 mRNA by quantitative RT–PCR analysis. (b) Luciferase mRNA (750 pg per cell) alone, NICD mRNA (250 pg per cell) plus Luciferase mRNA (500 pg per cell), or NICD mRNA (250 pg per cell) plus FoxJ1 mRNA (500 pg per cell) was injected into the animal region of the four blastomeres at the four-cell stage. Animal caps were isolated at stage 10. The animal caps were harvested at the equivalent of stage 19–20 and assayed for ERK7 mRNA by quantitative RT–PCR analysis. (c) Each MO (20 ng per cell) was injected into the four blastomeres at the four-cell stage. Animal caps were isolated at stage 10. The animal caps were harvested at the equivalent of stage 19–20 and assayed for ERK7 mRNA by quantitative RT–PCR analysis. Error bars represent the s.d. *P<0.05 by thet-test. Figure 3: ERK7 expression is under the control of FoxJ1. ( a – c ) Quantitative RT–PCR analysis of ERK7 expression levels. The average of three independent experiments is presented. The expression levels of ERK7 were normalized to those of ODC . ( a ) Each mRNA (500 pg per cell) was injected into the animal region of four blastomeres at the four-cell stage. Injected embryos were harvested at stage 13 and assayed for ERK7 mRNA by quantitative RT–PCR analysis. ( b ) Luciferase mRNA (750 pg per cell) alone, NICD mRNA (250 pg per cell) plus Luciferase mRNA (500 pg per cell), or NICD mRNA (250 pg per cell) plus FoxJ1 mRNA (500 pg per cell) was injected into the animal region of the four blastomeres at the four-cell stage. Animal caps were isolated at stage 10. The animal caps were harvested at the equivalent of stage 19–20 and assayed for ERK7 mRNA by quantitative RT–PCR analysis. ( c ) Each MO (20 ng per cell) was injected into the four blastomeres at the four-cell stage. Animal caps were isolated at stage 10. The animal caps were harvested at the equivalent of stage 19–20 and assayed for ERK7 mRNA by quantitative RT–PCR analysis. Error bars represent the s.d. * P <0.05 by the t -test. Full size image ERK7 is required for basal body migration in MCCs We determined the subcellular localization of ERK7. In MCCs, an ERK7-EGFP (enhanced green fluorescent protein) fusion protein was observed in a punctate pattern, suggesting the localization of ERK7 in the base of the cilia ( Fig. 4a ). In addition, ERK7 localized to cell–cell junctions ( Fig. 4a ) and weakly to cilia ( Supplementary Fig. 8a ). EGFP did not specifically localize to these regions ( Supplementary Fig. 8b ). Coexpression of ERK7-EGFP with Centrin2-mCherry (a basal body marker) showed that ERK7 localization overlapped with Centrin2 localization and was adjacent to a basal body ( Fig. 4b ). Coexpression of ERK7-EGFP with CLAMP-mCherry (a marker for striated ciliary rootlet) showed that ERK7 also localized to the striated ciliary rootlet ( Fig. 4c ). 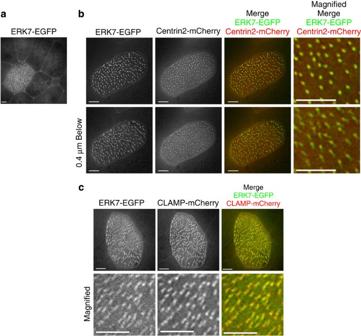Figure 4: Subcellular localization of ERK7 in MCCs. (a) Subcellular localization of ERK7-EGFP in the epidermis. ERK7-EGFP mRNA (25 pg per cell) was injected into the animal region of four blastomeres at the four-cell stage, and the injected embryos were observed at stage 33/34. (b) Subcellular localization of ERK7-EGFP (green) and Centrin2-mCherry (red) in the MCCs. ERK7-EGFP mRNA (25 pg per cell) and Centrin2-mCherry mRNA (50 pg per cell) were injected into the ventral marginal region of two blastomeres at the four-cell stage, and the injected embryos were observed at stage 35/36. (c) Subcellular localization of ERK7-EGFP (green) and CLAMP-mCherry (red) in the MCCs. ERK7-EGFP mRNA (25 pg per cell) and CLAMP-mCherry mRNA (100 pg per cell) were injected into the ventral two blastomeres at the four-cell stage, and the injected embryos were fixed at stage 33/34 and observed. Data are representative of two independent experiments. Scale bars, 5 μm. Figure 4: Subcellular localization of ERK7 in MCCs. ( a ) Subcellular localization of ERK7-EGFP in the epidermis. ERK7-EGFP mRNA (25 pg per cell) was injected into the animal region of four blastomeres at the four-cell stage, and the injected embryos were observed at stage 33/34. ( b ) Subcellular localization of ERK7-EGFP (green) and Centrin2-mCherry (red) in the MCCs. ERK7-EGFP mRNA (25 pg per cell) and Centrin2-mCherry mRNA (50 pg per cell) were injected into the ventral marginal region of two blastomeres at the four-cell stage, and the injected embryos were observed at stage 35/36. ( c ) Subcellular localization of ERK7-EGFP (green) and CLAMP-mCherry (red) in the MCCs. ERK7-EGFP mRNA (25 pg per cell) and CLAMP-mCherry mRNA (100 pg per cell) were injected into the ventral two blastomeres at the four-cell stage, and the injected embryos were fixed at stage 33/34 and observed. Data are representative of two independent experiments. Scale bars, 5 μm. Full size image Ciliogenesis is a multistep process [7] . During ciliogenesis, basal bodies are formed either from pre-existing centrioles or de novo . After formation, basal bodies migrate apically and nucleate axonemal microtubules. To investigate the behaviour of basal bodies, we performed immunostaining with a γ-tubulin antibody. In control embryos, basal bodies of MCCs were located apically and docked at the apical membrane ( Fig. 5a ), as previously reported [11] . However, in ERK7 morphants, most of basal bodies failed to migrate apically and remained located deep within the cytoplasm ( Fig. 5a ). This mislocalization of basal bodies in ERK7 morphants was more clearly visualized in transverse sections ( Fig. 5b ). These results indicate that ERK7 is required for basal body migration in MCCs. 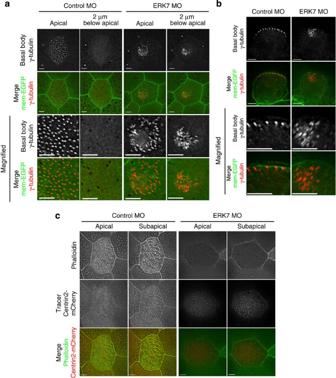Figure 5: ERK7 is required for basal body migration. (a–c) Each MO (15 ng per cell) was injected into the ventral marginal region of two blastomeres at the four-cell stage, and the embryos were fixed at stage 35/36. (a,b) MCCs of embryos immunostained with anti-γ-tubulin to visualize basal bodies (red). As a tracer, mem-EGFP (green) was used. (b) Transverse sections of the embryos shown ina. (c) MCCs of embryos stained with phalloidin to visualize actin meshworks (green). MCCs were detected by multipunctate localization of Centrin2-mCherry (red). Data are representative of two independent experiments. Scale bars, 5 μm. Figure 5: ERK7 is required for basal body migration. ( a – c ) Each MO (15 ng per cell) was injected into the ventral marginal region of two blastomeres at the four-cell stage, and the embryos were fixed at stage 35/36. ( a , b ) MCCs of embryos immunostained with anti-γ-tubulin to visualize basal bodies (red). As a tracer, mem-EGFP (green) was used. ( b ) Transverse sections of the embryos shown in a . ( c ) MCCs of embryos stained with phalloidin to visualize actin meshworks (green). MCCs were detected by multipunctate localization of Centrin2-mCherry (red). Data are representative of two independent experiments. Scale bars, 5 μm. Full size image In Xenopus MCCs, two distinct pools of actin, apical actin and subapical actin, form actin meshworks at the apical surface [29] . It has previously been shown that the apical actin meshwork is important for basal body migration [11] , [30] , [31] . Phalloidin staining in MCCs showed that knockdown of ERK7 caused a drastic loss of both the apical and subapical actin meshwork ( Fig. 5c ). These results strongly suggest that ERK7 regulates basal body migration by organizing the actin meshwork. ERK7 phosphorylates CapZIP To examine the molecular mechanisms by which ERK7 regulates ciliogenesis and actin organization, we searched for a direct substrate of ERK7 in ciliogenesis. CapZIP emerged as a potential substrate of ERK7 based on the following previous observations: (1) CapZIP has been shown to regulate ciliogenesis in a phosphorylation-dependent manner [10] ; (2) the phosphorylation sites essential for CapZIP function in ciliogenesis coincide with MAP kinase consensus sequences; and (3) CapZIP regulates actin formation [10] . CapZIP was originally identified as a substrate for MAPKAP-K2, p38γ and p38δ in skeletal muscle [32] , but it remains unknown which kinase phosphorylates CapZIP during ciliogenesis. Therefore, we hypothesized that ERK7 would regulate ciliogenesis by phosphorylating CapZIP. To investigate whether ERK7 phosphorylates CapZIP, we first performed coexpression experiments. Coexpression of CapZIP with ERK7, but not with a kinase-dead ERK7 mutant (ERK7 KD), caused a mobility shift of CapZIP, which suggested that ERK7 phosphorylates CapZIP ( Fig. 6a ). Xenopus CapZIP has nine MAP kinase consensus sequences (serine/threonine followed by proline) ( Supplementary Fig. 9 ). Of the nine residues, six are well conserved among mouse, human and Xenopus . Of the six residues, two serine residues (S81 and S108 in Xenopus CapZIP) have been reported to be important for the function of CapZIP during ciliogenesis [10] . Therefore, we generated two CapZIP mutants: CapZIP 2A and CapZIP 6A. In CapZIP 2A, the two reported residues were replaced with alanine, and in CapZIP 6A, the six conserved residues were replaced with alanine. When coexpressed with ERK7, the mobility of the shifted bands of CapZIP 2A was much faster than that of CapZIP WT ( Fig. 6a ), and CapZIP 6A produced no mobility shifted bands ( Fig. 6a ). Thus, it is likely that ERK7 phosphorylates CapZIP at several of these six residues, including the two residues. 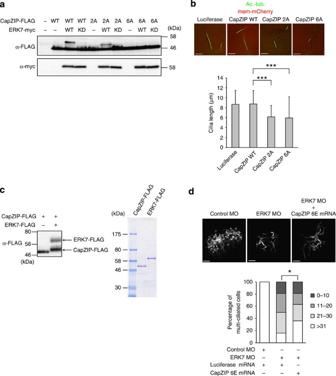Figure 6: ERK7 phosphorylates CapZIP. (a) Immunoblotting analysis of the phosphorylation status of CapZIP in lysates from HEK293T cells transfected with the indicated combinations of expression vectors. (b) Cilia (green) on the GRP. Each mRNA (1.5 ng per cell) was injected with mem-mCherry (red) mRNA into the dorsal marginal region of two blastomeres at the four-cell stage. The lower graph shows the average length of cilia on the GRP (luciferase,n=30 from five dorsal explants; CapZIP WT,n=84 from five dorsal explants; CapZIP 2A,n=82 from six dorsal explants; CapZIP 6A,n=19 from three dorsal explants). Scale bars, 5 μm. Error bars represent the s.d. ***P<0.001 by thet-test. (c)In vitrokinase assays using purified ERK7 and CapZIP proteins. FLAG-CapZIP and FLAG-ERK7 were expressed separately in HEK293T cells, and purified as shown by Coomassie brilliant blue staining (right panel). (d) The indicated sets of MO (10 ng per cell), luciferase or CapZIP 6E mRNA (1 ng per cell) and Centrin2-EGFP mRNA (100 pg per cell) were injected into the ventral marginal region of one blastomere at the four-cell stage. Centrin2-EGFP was used as a tracer. The injected embryos were harvested at stage 35/36 and immunostained with anti-acetylated α-tubulin. The number of cilia in MCCs (n=100) from 10 embryos of two independent experiments for each condition was scored. Representative images of MCCs are shown for each condition. Scale bars, 5 μm. *P<0.05 by the Mann–WhitneyU-test. Figure 6: ERK7 phosphorylates CapZIP. ( a ) Immunoblotting analysis of the phosphorylation status of CapZIP in lysates from HEK293T cells transfected with the indicated combinations of expression vectors. ( b ) Cilia (green) on the GRP. Each mRNA (1.5 ng per cell) was injected with mem-mCherry (red) mRNA into the dorsal marginal region of two blastomeres at the four-cell stage. The lower graph shows the average length of cilia on the GRP (luciferase, n =30 from five dorsal explants; CapZIP WT, n =84 from five dorsal explants; CapZIP 2A, n =82 from six dorsal explants; CapZIP 6A, n =19 from three dorsal explants). Scale bars, 5 μm. Error bars represent the s.d. *** P <0.001 by the t -test. ( c ) In vitro kinase assays using purified ERK7 and CapZIP proteins. FLAG-CapZIP and FLAG-ERK7 were expressed separately in HEK293T cells, and purified as shown by Coomassie brilliant blue staining (right panel). ( d ) The indicated sets of MO (10 ng per cell), luciferase or CapZIP 6E mRNA (1 ng per cell) and Centrin2-EGFP mRNA (100 pg per cell) were injected into the ventral marginal region of one blastomere at the four-cell stage. Centrin2-EGFP was used as a tracer. The injected embryos were harvested at stage 35/36 and immunostained with anti-acetylated α-tubulin. The number of cilia in MCCs ( n =100) from 10 embryos of two independent experiments for each condition was scored. Representative images of MCCs are shown for each condition. Scale bars, 5 μm. * P <0.05 by the Mann–Whitney U -test. Full size image CapZIP has been shown to be essential for ciliogenesis in zebrafish, and phosphorylation of CapZIP on the two serine residues is important for its function [10] . We next examined the expression patterns of CapZIP during early Xenopus development by quantitative RT–PCR and whole-mount in situ hybridization. Quantitative RT–PCR experiments showed that CapZIP expression was detected at stage 12 (late gastrula stage) and thereafter, and then gradually increased until stage 25 (early tailbud stage; Supplementary Fig. 10a ). Whole-mount in situ hybridization experiments showed that CapZIP was expressed in the DIMZ at stage 14 ( Supplementary Fig. 10b ) and in the epidermis at stages 14, 17 and 23 ( Supplementary Fig. 10b–d ), indicating that CapZIP and ERK7 are expressed in overlapping regions. CapZIP expression was also detected in the somites and heart field ( Supplementary Fig. 10d,e ). Next, we examined whether the roles of CapZIP and its phosphorylation in ciliogenesis are conserved in Xenopus . Injection of CapZIP 2A mRNA, but not CapZIP WT mRNA, resulted in a significant reduction in the length of cilia in the GRP ( Fig. 6b and Supplementary Fig. 10f ). CapZIP 6A expression had the same effect on the length of cilia as CapZIP 2A ( Fig. 6b and Supplementary Fig. 10f ). These results indicate that CapZIP also regulates ciliogenesis in a manner that is dependent on its phosphorylation at S81 and S108 in Xenopus . To investigate whether ERK7 directly phosphorylates CapZIP, we performed an in vitro kinase assay using purified FLAG-tagged ERK7 and FLAG-tagged CapZIP. The incubation of these two proteins in the presence of ATP produced mobility shifted bands of CapZIP ( Fig. 6c ), indicating that ERK7 directly phosphorylates CapZIP. To provide evidence for the functional significance, we next examined whether the expression of a phosphomimetic mutant of CapZIP rescues the ciliogenesis defect in the ERK7 morphants. To achieve this goal, we made a CapZIP 6E mutant, in which the six conserved residues were replaced with glutamic acid. The injection of CapZIP 6E mRNA significantly rescued the defect in cilia formation in ERK7 morphants ( Fig. 6d ), indicating that ERK7-mediated phosphorylation of CapZIP is important for ciliogenesis in vivo . Dvl facilitates ERK7 phosphorylation of CapZIP CapZIP has been shown to be a non-canonical Wnt signalling mediator and to function downstream of Dvl [10] . Remarkably, the knockdown phenotypes and the subcellular localization pattern of Dvl in MCCs [11] are similar to those of ERK7. Knockdown of Dvl leads to a failure of basal body migration and loss of the apical actin meshwork in Xenopus MCCs [11] , and the subcellular localization of Dvl2, which localized near basal bodies in MCCs, is important for ciliogenesis [11] . In addition, we found that overexpression of ERK7 resulted in a severely shortened anterior–posterior axis ( Supplementary Fig. 11a ), and the phenotype is related to the function of Dvl [33] , [34] . These observations prompted us to investigate the relationship between ERK7 and Dvl. First, to examine whether ERK7 co-localizes with Dvl2 in MCCs, we coinjected Dvl2-EGFP and ERK7-mCherry mRNAs. As previously reported [11] , Dvl2-EGFP localized both at smaller foci (near the basal bodies) and at larger aggregates in MCCs ( Fig. 7a and Supplementary Fig. 11b ). ERK7-mCherry co-localized with Dvl2-EGFP at smaller foci and partly at larger aggregates. These results suggest that ERK7 and Dvl2 would form a complex. To test this idea, we performed coimmunoprecipitation assays in cultured cells and found that Dvl2 coimmunoprecipitated with ERK7 ( Fig. 7b ) and vice versa ( Supplementary Fig. 11c ). Our results also showed coimmunoprecipitation of mouse ERK7 with mouse Dvl2 ( Supplementary Fig. 11d ). 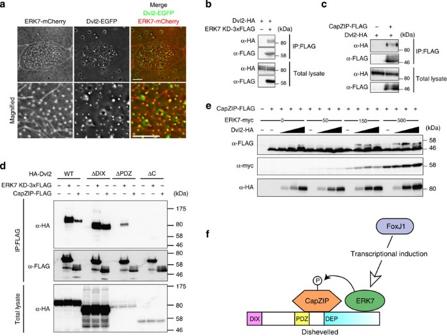Figure 7: Dvl facilitates ERK7-mediated phosphorylation of CapZIP through binding to both ERK7 and CapZIP. (a) The subcellular localization of ERK7-mCherry (red) and Dvl2-EGFP (green) in MCCs. ERK7-mCherry mRNA (50 pg per cell) and Dvl2-EGFP mRNA (100 pg per cell) were injected into the ventral marginal region of two blastomeres at the four-cell stage, and the embryos were observed at stage 25. Scale bars, 5 μm. (b–d) Coimmunoprecipitation assays using lysates from HEK293T cells transfected with the indicated combinations of expression vectors. To prevent the dissociation of a substrate from a kinase upon phosphorylation, we used a kinase-dead mutant of ERK7. (b) Coimmunoprecipitation of ERK7 with Dvl2. (c) Coimmunoprecipitation of CapZIP with Dvl2. (d) Coimmunoprecipitation of ERK7 or CapZIP with a series of Dvl2 deletion mutant. (e) Immunoblotting analysis of ERK7-mediated phosphorylation of CapZIP in the presence of increasing amounts of Dvl2. The indicated combinations of expression vectors were transfected into HEK293T cells. (f) Model for ERK7 action. Data are representative of two independent experiments. Figure 7: Dvl facilitates ERK7-mediated phosphorylation of CapZIP through binding to both ERK7 and CapZIP. ( a ) The subcellular localization of ERK7-mCherry (red) and Dvl2-EGFP (green) in MCCs. ERK7-mCherry mRNA (50 pg per cell) and Dvl2-EGFP mRNA (100 pg per cell) were injected into the ventral marginal region of two blastomeres at the four-cell stage, and the embryos were observed at stage 25. Scale bars, 5 μm. ( b – d ) Coimmunoprecipitation assays using lysates from HEK293T cells transfected with the indicated combinations of expression vectors. To prevent the dissociation of a substrate from a kinase upon phosphorylation, we used a kinase-dead mutant of ERK7. ( b ) Coimmunoprecipitation of ERK7 with Dvl2. ( c ) Coimmunoprecipitation of CapZIP with Dvl2. ( d ) Coimmunoprecipitation of ERK7 or CapZIP with a series of Dvl2 deletion mutant. ( e ) Immunoblotting analysis of ERK7-mediated phosphorylation of CapZIP in the presence of increasing amounts of Dvl2. The indicated combinations of expression vectors were transfected into HEK293T cells. ( f ) Model for ERK7 action. Data are representative of two independent experiments. Full size image Given that Dvl functions as a scaffold by providing a signalling platform in diverse contexts [35] , we hypothesized that Dvl should facilitate ERK7 phosphorylation of CapZIP by serving as a scaffold. To examine this possibility, we first investigated whether Dvl binds to CapZIP. Coimmunoprecipitation experiments showed that Dvl2 binds to CapZIP ( Fig. 7c ). Next, by using a series of Dvl2 deletion mutants, we determined an ERK7-binding site and a CapZIP-binding site in Dvl2. ERK7 coimmunoprecipitated with Dvl2 WT, Dvl2 ΔDIX (a deletion mutant of the DIX domain) and Dvl2 ΔPDZ (a deletion mutant of the PDZ domain), but not with Dvl2 ΔC (a deletion mutant of the C-terminal region containing the DEP domain; Fig. 7d ). CapZIP coimmunoprecipitated with Dvl2 WT and Dvl2 ΔDIX, but not with Dvl2 ΔPDZ or Dvl2 ΔC. These results indicate that ERK7 and CapZIP bind to Dvl2 at the C-terminal region and at the region spanning both the PDZ domain and the C-terminal region, respectively ( Fig. 7f ). Finally, to examine whether Dvl2 could enhance ERK7 phosphorylation of CapZIP, we examined the effect of increasing amounts of Dvl2 on ERK7-mediated phosphorylation of CapZIP. The data show that the phosphorylation of CapZIP was enhanced by increasing the concentration of Dvl2, but the extent of phosphorylation tended to decrease when the concentration of Dvl2 became too high ( Fig. 7e ). This biphasic nature of the effect of its increasing concentrations is a well-known characteristic of the action of a scaffold protein. Thus, these results taken together indicate that Dvl2 functions as a scaffold in ERK7-mediated phosphorylation of CapZIP ( Fig. 7f ). Mouse ERK7 is involved in ciliogenesis We finally investigated whether the role of ERK7 in ciliogenesis is conserved in mammals. To achieve this goal, we used mouse tracheal epithelial cells (mTECs), in which ciliogenesis is triggered by exposure to an air–liquid interface (ALI) [36] . It has been previously established that MCCs start to be induced at ~3–4 days after exposure of confluent mTECs to ALI [37] . First, we examined the changes in gene expression during ciliogenesis in mTECs. ERK7 mRNA exhibited peak expression at ~5 days after ALI exposure, whereas the expression of FoxJ1 was initiated earlier and peaked at ~2 days after ALI exposure ( Fig. 8a ). This result is consistent with our hypothesis that ERK7 expression is under the control of FoxJ1 . Dnah9, Tekt2, Spag6 and Rsph1 (also known as radial spoke protein 44) are present in axonemal structures exclusive to motile cilia and are known to be upregulated by FoxJ1 (refs 12 , 25 ). These four genes also exhibited peak expression of ~5 days after ALI exposure, similarly to ERK7 expression ( Fig. 8a ). 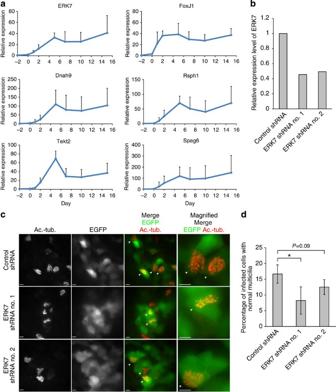Figure 8: ERK7 plays a role in ciliogenesis in mTECs. (a) Quantitative RT–PCR analysis ofERK7,FoxJ1,Dnah9,Rsph1,Tekt2andSpag6expression levels during the time course of mTEC differentiation. The average of three (ALI+1) or four (ALI-2, 0, +2, +5, +7, +10 and +15) independent experiments is shown. Error bars represent the s.d. (b) Knockdown efficiency of shRNA constructs against mouseERK7was assessed using mIMCD3 cells. (c,d) Knockdown of ERK7 in mTECs using lentivirus vectors encoding shRNA. At 8 days after ALI creation, mTECs were fixed for immunostaining with anti-acetylated α-tubulin (Ac.-tub.) to visualize cilia (red). EGFP (green) indicates infected cells. (d) The percentage of infected cells with normal multicilia (arrowhead inc) among all of the infected cells was calculated by counting the cell number in thirty fields (at least 500 cells for each condition were assessed). The average of three independent experiments is shown. *P<0.05. Statistical significance was determined by thet-test. Error bars represent the s.d. Scale bars, 5 μm. Figure 8: ERK7 plays a role in ciliogenesis in mTECs. ( a ) Quantitative RT–PCR analysis of ERK7 , FoxJ1 , Dnah9 , Rsph1 , Tekt2 and Spag6 expression levels during the time course of mTEC differentiation. The average of three (ALI+1) or four (ALI-2, 0, +2, +5, +7, +10 and +15) independent experiments is shown. Error bars represent the s.d. ( b ) Knockdown efficiency of shRNA constructs against mouse ERK7 was assessed using mIMCD3 cells. ( c , d ) Knockdown of ERK7 in mTECs using lentivirus vectors encoding shRNA. At 8 days after ALI creation, mTECs were fixed for immunostaining with anti-acetylated α-tubulin (Ac.-tub.) to visualize cilia (red). EGFP (green) indicates infected cells. ( d ) The percentage of infected cells with normal multicilia (arrowhead in c ) among all of the infected cells was calculated by counting the cell number in thirty fields (at least 500 cells for each condition were assessed). The average of three independent experiments is shown. * P <0.05. Statistical significance was determined by the t -test. Error bars represent the s.d. Scale bars, 5 μm. Full size image We next designed mouse ERK7 short hairpin RNA (shRNA) constructs (nos. 1 and 2) and confirmed that these shRNA sequences effectively suppressed ERK7 expression in mIMCD3 cells ( Fig. 8b ). To investigate the function of ERK7 in the ciliogenesis of mTECs, we introduced our ERK7 shRNA constructs using lentivirus. While ~17% of mTECs expressing control shRNA formed mature multicilia, the proportion of mTECs with mature multicilia was reduced to ~8% by ERK7 shRNA ( Fig. 8c,d ). These results show that ERK7 plays a role in ciliogenesis in mammals. In this study, we identified ERK7 as a key regulator of ciliogenesis. In addition, we showed that ERK7 expression is under the control of FoxJ1 . Because ERK7 is constitutively active [3] , the regulation at the expression level should be crucial for ERK7 function. It has been previously shown that knockdown of FoxJ1, similarly to knockdown of ERK7, results in a failure in basal body migration and a loss of the actin meshwork in MCCs [12] . Thus, our results strongly suggest that FoxJ1 regulates actin organization and basal body migration at least in part through the induction of ERK7. Knockdown of ERK7 resulted in reduced head structures. Because Wnt signalling is known to be important for head formation [38] , there may be a link between ERK7 and Wnt signalling. Interestingly, FoxJ1 expression has been shown to be regulated by canonical Wnt signalling [39] , [40] . Thus, a canonical Wnt signalling pathway may regulate ERK7 expression levels through FoxJ1 . Dvl regulates various biological processes, including ciliogenesis [11] , and it has various modes of action that are achieved with different interaction partners [35] . Our findings demonstrate that Dvl regulates the efficiency of ERK7-mediated phosphorylation of CapZIP, which has been shown to regulate ciliogenesis in a phosphorylation-dependent manner [10] , by binding to both ERK7 and CapZIP. In addition, knockdown of ERK7 disturbed the polarization of GRP cilia. Interestingly, non-canonical Wnt signalling regulates the polarization of cilia in Xenopus GRP, mouse node and zebrafish Kuppfer’s vesicle [41] , [42] , [43] , [44] . CapZIP has been shown to be a non-canonical Wnt signalling mediator that functions downstream of Dvl [10] , and thus, ERK7 should play a crucial role in linking the FoxJ1-induced ciliogenesis programme to non-canonical Wnt signalling. Embryo manipulations Xenopus embryos were obtained by in vitro fertilization and cultured in 0.1 × modified Barth's saline (MBS) (1.0 mM HEPES (pH 7.4), 8.8 mM NaCl, 0.1 mM KCl, 0.24 mM NaHCO 3 , 0.082 mM MgSO 4 , 0.03 mM Ca(NO 3 ) 2 and 0.041 mM CaCl 2 ). Embryos injections were performed in 4% Ficoll in 0.1 × MBS. Frogs were bred and handled with care, according to the established manual [45] . The in vitro synthesis of capped mRNA was performed using mMESSAGE mMACHINE (Ambion) according to the manufacturer’s instructions. Antisense MOs were obtained from Gene Tools, Inc. The MO sequences were as follows: ERK7 MO, 5′-ATCTTCCACCTCTGGGCCACTCATG-3′; second non-overlapping ERK7 MO, 5′-ATGTCACACAACAACTGGCCCCTCC-3′; FoxJ1 MO (described as XFoxJ1-MOATG in previous study [12] ), 5′-GCAGGTCAAACATTAATAAAGCCCT-3′ and a standard control oligo (control MO), 5′-CCTCTTACCTCAGTTACAATTTATA-3′. To assess cilium formation in the GRP, dorsal explants were dissected at stage 16, and placed underneath a glass coverslip with silicone vacuum grease. To monitor the hovering movement of embryos, we anaesthetized embryos with MS-222 (Sigma) on agar plates. First, the embryo was placed on the uninjected left side, and then, it was flipped to the injected right side as described in a previous study [46] . To assess the fluid flow, we immobilized anaesthetized embryos at stage 33/34 in 1% Steinberg agar plates and added fluorescent beads (F8844, Invitrogen) to the culture media. To measure the flow velocity of the beads, 10 beads were chosen from the beads above an embryo at random and the flow speed was measured using ImageJ. Images and movies were acquired using the stereomicroscope SZX12 (Olympus) equipped with the digital camera DP50 (Olympus), SZX16 (Olympus) equipped with the digital camera DP73 (Olympus) or the Delta Vision optical sectioning system (Applied Precision) equipped with the inverted microscope IX71 (Olympus), the charge-coupled device camera CoolSNAP HQ Monochrome (Photometrics) and SoftWoRx software (Applied Precision). Image deconvolution was performed using SoftWoRx software. To display the trajectories of the fluorescent beads, movies of the bead movement were processed as follows, which was modified from a previous study [13] : (1) each frame of the movie was converted to a binary image and then applied to Watershed segmentation using ImageJ; and (2) each of the frames was assigned a pseudocolour ranging from yellow (frame 1, time 0 s) to red (frame 33, time 3.3 s), and all of the frames were merged using Adobe Photoshop CS5 (Adobe Systems). Molecular cloning and plasmid construction The entire coding region of Xenopus laevis ERK7 (NM_001095966), X. laevis FoxJ1 (AJ609390), X. laevis CapZIP (AB920341), X. laevis Centrin2 (NM_001096664), X. laevis CLAMP (NM_001096937), mouse ERK7 (NM_177922) and mouse Dvl2 (NM_007888) were amplified using PCR and cloned into the expression vector. To obtain a kinase-negative form of ERK7 (ERK7 KD), Lys43 in X. laevis ERK7 and Lys43 in mouse ERK7 were replaced with arginines. To obtain the CapZIP 2A mutant, Ser81 and Ser108 were replaced with alanines. To obtain the CapZIP 6A mutant, Ser81, Ser108, Ser116, Ser120, Thr124 and Ser127 were replaced with alanines. To obtain the CapZIP 6E mutant, Ser81, Ser108, Ser116, Ser120, Thr124 and Ser127 were replaced with glutamic acids. All of the Xenopus CapZIP constructs were cloned into the FLAG-tagged pCS2+ expression vector. The deletion mutant series of X. laevis Dvl2 was inserted into the hemagglutinin (HA)-tagged pCS2+ expression vector [47] . To obtain membrane-targeted mCherry and EGFP, the human K-Ras C-terminal 18 amino acids were fused to mCherry and EGFP, respectively. To generate an ERK7 MO-resistant construct for the rescue experiments, nine silent mutations were introduced into the MO target sequence of X. laevis ERK7 by site-directed mutagenesis, which replaces 5′-CATGAGTGGCCCAGAGGTGGAAGAT-3′ with 5′-CATG TCA GG G CC T GA A GT C GA G GA C -3′ (underlines indicate mutated nucleotides). Amino-acid sequence alignment was performed using GENETYX software (Genetyx Corp.). Whole-mount in situ hybridization and immunostaining Whole-mount in situ hybridization was performed according to the standard protocol [45] using a robot (InsituPro, Intavis). Briefly, embryos were fixed in MEMFA (100 mM MOPS (pH 7.4), 2 mM EGTA, 1 mM MgSO 4 and 3.7% formaldehyde) and dehydrated in methanol. After rehydration, embryos were treated with 5 μg ml −1 proteinase K in PBS containing 0.1% Tween20, incubated in 100 mM triethanolamine (pH 8.0), incubated in 100 mM triethanolamine containing 0.25% acetic anhydride and then refixed with 4% paraformaldehyde in PBS. After washing, embryos were hybridized with RNA probes and then subjected to anti-digoxigenin antibody staining (no. 11093274910, Roche; 1:2,000). The colour reaction was performed using BM purple. For double in situ hybridization, the first colour reaction was performed using BM purple. To inactivate remaining alkaline phosphatase derived from the first reaction, stained embryos were incubated with the maleic acid buffer (100 mM maleic acid (pH 7.5) and 150 mM NaCl) containing 10 mM EDTA at 65 °C for 15 min, and dehydrated in methanol. After rehydration, embryos were refixed with 4% paraformaldehyde in PBS, and then subjected to anti-fluorescein antibody staining (no. 11426338910, Roche; 1:4,000). The second colour reaction was performed using 5-bromo-4-chloro-3-indolyl phosphate (BCIP). The following digoxigenin-labelled RNA probes were used: X. laevis ERK7 (the entire coding region of NM_001095966), X. laevis tph1 (the entire coding region of NM_001087454), X. laevis Pitx2c (the entire region of AJ243596) and X. laevis CapZIP (bp 601–978 of AB920341). The fluorescein-labelled RNA probe of FoxJ1 was synthesized from the cDNA corresponding to the coding region of X. laevis FoxJ1 (AJ609390). For in situ hybridization followed by immunostaining, we omitted the proteinase K step. Immunostaining procedures for Xenopus embryos were modified from previously described methods [48] . Briefly, the embryos were fixed in 4% paraformaldehyde in PBS for 2 h at room temperature or overnight at 4 °C. For γ-tubulin immunostaining, the embryos were dehydrated in Dent’s fixative. Fixed embryos were washed with PBS containing 0.1% Triton X-100 (PBT) and blocked with 10% fetal bovine serum (FBS) and 5% dimethylsulphoxide in PBT for 1 h. Embryos were incubated with primary antibodies at 4 °C overnight. After washing five times with PBT for 1 h, the embryos were incubated with the appropriate secondary antibodies at 4 °C overnight followed by washing with PBT. The following antibodies were used at the indicated dilutions. The primary antibodies were mouse anti-acetylated α-tubulin (T7451, Sigma; 1:1,000), rabbit anti-GFP (A-11122, Invitrogen; 1:1,000) and mouse anti-γ-tubulin (T5236, Sigma; 1:500). The secondary antibodies were Alexa Fluor 350-conjugated anti-mouse IgG (A-21049, Invitrogen; 1:500), Alexa Fluor 488-conjugated anti-mouse IgG (A-11029, Invitrogen; 1:500), Alexa Fluor 488-conjugated anti-rabbit IgG (A-11034, Invitrogen; 1:500) and Alexa Fluor 568-conjugated anti-mouse IgG (A-11031, Invitrogen; 1:500). To visualize actin, we used Alexa Fluor 488-conjugated phalloidin (Invitrogen). The length of the cilia was measured with SoftWoRx software. For cryosectioning, embryos were washed with PBS, and embedded in 7.5% gelatin and 15% sucrose in PBS. The embedded embryos were frozen in liquid N 2 and sectioned at 10 μm using a Microm HM500 OM microtome cryostat (CarlZeiss). For immunostaining of mTECs, cells were fixed in 4% paraformaldehyde at room temperature for 10 min and then submerged in cold methanol for 5 min at −20 °C. After blocking with 3% bovine serum albumin in PBS at room temperature for 30 min, cells were incubated with 3% bovine serum albumin in PBS containing the primary antibody at 4 °C overnight, washed with PBS and then incubated with the appropriate secondary antibodies for 30 min at room temperature. Finally, the cells were mounted in Mowiol. Cell culture and transfection HEK293T and mIMCD3 cells were obtained from the American Type Culture Collection. HEK293T cells were cultured in Dulbecco’s modified Eagle’s medium (DMEM) containing 10% FBS. mIMCD3 cells were cultured in DMEM/F12 containing 10% FBS. HEK293T cells were cultured on collagen-coated plates. Cells were transfected using Lipofectamine 2000 (Invitrogen) or Fugene HD (Promega) according to the manufacturer’s protocol. Immunoprecipitation and immunoblotting Embryos or cells were lysed in Lysis buffer (20 mM Tris-Cl (pH 7.5), 150 mM NaCl, 1.5 mM MgCl 2 , 2 mM EGTA, 25 mM β-glycerophosphate, 10 mM sodium pyrophosphate, 1% NP-40, 10 mM NaF, 2 mM dithiothreitol and 1 mM phenylmethylsulphonyl fluoride) or immunoprecipitation (IP) buffer for co-IP (20 mM HEPES (pH 7.8), 100 mM NaCl, 1.5 mM MgCl 2 , 1 mM EGTA, 10 mM sodium pyrophosphate, 1% NP-40, 10% glycerol and 1 mM phenylmethylsulphonyl fluoride) containing protease inhibitor cocktail (Sigma) and PhosSTOP phosphatase inhibitor cocktail (Roche). Anti-FLAG M2 affinity gel (Sigma) was used for immunoprecipitation of FLAG-tagged proteins. Protein G-Sepharose beads (GE Healthcare) and an anti-HA antibody (16B12, 1:300; Covance) were used for immunoprecipitation of HA-tagged proteins. The precipitates were washed three times with Lysis buffer or IP buffer and then subjected to elution by boiling with Laemmli’s sample buffer, or by adding 3 × FLAG peptide (Sigma) or ERK7 peptide. The samples were resolved by SDS–PAGE and subjected to immunoblotting according to a standard protocol. Signals were usually detected with Western Lightning Plus-ECL Enhanced Chemiluminescence reagent (PerkinElmer). ECL prime (GE Healthcare) was used to detect signals for endogenous ERK7. The following antibodies were used at the indicated dilutions. The primary antibodies were mouse anti-Myc (9E10, 1:2,000; Santa Cruz Biotechnology), mouse anti-FLAG (M2, 1:4,000; Sigma), mouse anti-HA (16B12, 1:1,000; Covance), mouse anti-α-tubulin (DM1A, 1:20,000; Sigma) and rabbit anti-ERK7 (1:2,000). The secondary antibodies were sheep anti-mouse IgG horseradish peroxidase (HRP)-conjugated (NA9310, 1:10,000; GE Healthcare) and donkey anti-rabbit IgG HRP-conjugated (NA9340, 1:10,000 for Western Lightning Plus-ECL, 1:100,000 for ECL prime; GE Healthcare). Some membranes were stripped using the Restore PLUS Western Blot Stripping buffer (Thermo Scientific) and reprobed with another antibody. Uncropped images of blots are shown in Supplementary Figs 12 and 13 . Antibody production and affinity purification The anti-ERK7 polyclonal antibody was produced in rabbits by immunizing them with a synthetic peptide corresponding to residues 414–430 of Xenopus ERK7 (QKDSTQQSPKIKAPSSN) plus an additional N-terminal cysteine for conjugation. Rabbit antisera were affinity purified using the synthetic peptide. The antibody was dialysed and concentrated. The peptide synthesis, immunizations and affinity purification were performed by MBL Co. Kinase assays For protein preparations, FLAG-tagged ERK7 and FLAG-tagged CapZIP were expressed separately in HEK293T cells, precipitated by anti-FLAG M2 affinity gel (Sigma), and eluted using 3 × FLAG peptide. For the kinase assays, FLAG-tagged ERK7 protein was mixed with FLAG-tagged CapZIP protein in a kinase reaction buffer (50 mM Tris-Cl (pH 7.5), 0.1 mM EGTA, 10 mM magnesium acetate, 0.1 mM sodium orthovanadate and 1 mM ATP), which was modified from a previous study [49] , and incubated for 30 min at 30 °C. The reactions were stopped by addition of Laemmli’s sample buffer and boiling. Quantitative RT–PCR Total RNA from Xenopus embryos was extracted using TRIzol reagent (Invitrogen) and the cDNA was synthesized using M-MLV reverse transcriptase (Invitrogen). Total RNA extraction from mammalian cells was performed with the QIAGEN RNeasy Mini Kit (Qiagen), and the cDNA was synthesized using the QuantiTect Reverse Transcription Kit (Qiagen). Quantitative RT–PCR was performed with a 7300 real-time PCR System (Applied Biosystems) using SYBR Green PCR Master Mix (Qiagen). Duplicate PCRs were performed for each sample in each experiment. The gene expression levels were normalized to those of ODC in Xenopus embryos or GAPDH in mammalian cells. The primers used for quantitative RT–PCR were as follows: Xenopus ERK7 (forward 5′-AAAGCCATTGATCGCAAATC-3′; reverse 5′-GCTCGAATCACATTCAGCAA-3′); Xenopus ODC (forward 5′-TGCAAGTTGGAGACTGGATG-3′; reverse 5′-CATCAGTTGCCAGTGTGGTC-3′); Xenopus FoxJ1 (forward 5′-CCCCTGAGTCCAGTTACACG-3′; reverse 5′- TATTTTGCGCCACCGCATGA-3′); Xenopus CapZIP (forward 5′-TTCAGCAGTCCCCCATTGAC-3′; reverse 5′-ACTCTGTCAGGGATTTGCGG-3′); mouse ERK7 (forward 5′-GCCCGGACGCAATCGCTCAA-3′; reverse 5′-GGGCTACGCGGAGGTTTGGG-3′); mouse GAPDH (forward 5′-TGCGACTTCAACAGCAACTC-3′; reverse 5′-GCCTCTCTTGCTCAGTGTCC-3′); mouse FoxJ1 (forward 5′-CTCTGAGCCAGGCCTCACATT-3′; reverse 5′-GGTCAACATCCACAGGCTGA-3′); mouse Dnah9 (forward 5′-GGCCCCACATGGTATGTCAA-3′; reverse 5′-ACTGTGGCCATCCACAAACT-3′); mouse Rsph1 (forward 5′-ACGTAGACACGTTCAGGCAG-3′; reverse 5′-TAACTAAGGCACGCCTGGTG-3′); mouse Spag6 (forward 5′-CGCATACACAGAGGAACGGA-3′; reverse 5′-CCACCATCTGCACGAATTGC-3′); mouse Tekt2 (forward 5′-TTCGGCAGCAACTCAACTCT-3′; reverse 5′-GACGCTTTCATTTCGGCCTC-3′). Preparation of lentiviral vectors Constructs expressing shRNAs against mouse ERK7 were generated by subcloning the silencing oligonucleotides into the ApaI/EcoRI site of the CSII-U6-MCS-EGFP vector, which was designed to coexpress shRNA and the EGFP reporter [50] . The sequences of the silencing oligonucleotides were as follows: ERK7 shRNA no. 1 sense, 5′-CGAAGGATGTTTGGCATCTTTCAAGAGAAGATGCCAAACATCCTTCGGCTTTTT-3′; ERK7 shRNA no. 1 antisense, 5′-AATTAAAAAGCCGAAGGATGTTTGGCATCTTCTCTTGAAAGATGCCAAACATCCTTCGGGCC-3′; ERK7 shRNA no. 2 sense, 5′-GCCGAAGGATGTTTGGCATCTTTCAAGAGAAGATGCCAAACATCCTTCGGCTTTTT-3′; ERK7 shRNA no. 2 antisense, 5′-AATTAAAAAGCCGAAGGATGTTTGGCATCTTCTCTTGAAAGATGCCAAACATCCTTCGGCGGCC-3′. To produce the recombinant lentivirus, the shRNA-expressing CSII-U6-MCS-EGFP vector was co-transfected with pCAG-HIVgp and pCMV-VSV-G-RSV-Rev into HEK293T cells. Culture supernatants containing the virus were collected ~48 h after transfection. For infection to mTECs, the lentiviral supernatants were concentrated to achieve 10 7 –10 8 infectious units per millilitre using PEG-it Virus Precipitation solution (System Biosciences). Isolation and lentivirus infection of mTECs The isolation and culture of mTECs were performed according to the published protocol [36] , [51] . Briefly, mTECs isolated from tracheas of 7-week-old wild-type C57BL/6J male mice were seeded onto Transwell Clear permeable membranes (Corning, no. 3460) coated with rat-tail collagen and then cultured with mTEC plus medium [36] . After reaching confluency, the mTECs were exposed to ALI and cultured with mTEC basic medium [36] containing 2% Nu-Serum (Becton-Dickinson). For the knockdown experiments, mTECs were spin-infected with the shRNA-expressing lentivirus at 2 days after seeding and exposed to ALI after reaching confluency. All mouse experiments were conducted in accordance with the Regulation on Animal Experimentation at Kyoto University, and approved by the Animal Experimentation Committee of Kyoto University. Statistics The unpaired Student’s t -test with a two-tailed distribution and χ 2 -test were performed using EXCEL (Microsoft). The Mann–Whitney U -test was performed using SPSS Software (IBM). Accession codes: The sequence data of Xenopus laevis CapZIP were deposited in the DDBJ database under the accession number AB920341 . How to cite this article: Miyatake, K. et al. ERK7 regulates ciliogenesis by phosphorylating the actin regulator CapZIP in cooperation with Dishevelled. Nat. Commun. 6:6666 doi: 10.1038/ncomms7666 (2015).